Stress-induced phase transformation and optical coupling of silver nanoparticle superlattices into mechanically stable nanowires One-dimensional silver materials display unique optical and electrical properties with promise as functional blocks for a new generation of nanoelectronics. To date, synthetic approaches and property engineering of silver nanowires have primarily focused on chemical methods. Here we report a simple physical method of metal nanowire synthesis, based on stress-induced phase transformation and sintering of spherical Ag nanoparticle superlattices. Two phase transformations of nanoparticles under stress have been observed at distinct length scales. First, the lattice dimensions of silver nanoparticle superlattices may be reversibly manipulated between 0–8 GPa compressive stresses to enable systematic and reversible changes in mesoscale optical coupling between silver nanoparticles. Second, stresses greater than 8 GPa induced an atomic lattice phase transformation, which induced sintering of silver nanoparticles into micron-length scale nanowires. The nanowire synthesis mechanism displays a dependence on both nanoparticle crystal surface orientation and presence of particular grain boundaries to enable nanoparticle consolidation into nanowires. Silver (Ag) nanostructured materials such as nanoparticles, nanorods and nanowires exhibit size- and shape-dependent optical and electronic properties that enable a wide variety of applications in photocatalysis, nanoelectronics, phototherapy and imaging [1] , [2] . An ability to precisely tune the size and shape of silver nanostructures beyond the nanometre scale is essential for such applications, which has prompted extensive efforts to develop synthetic methods and processes to fabricate Ag nanostructures. Chemical methods are most frequently used to synthesize Ag nanostructures through redox reactions, either via electrochemical processes or using reducing agents. For an example, ‘dealloying’ is one effective chemical method to fabricate three-dimensional continuous metal nanostructures [3] , [4] , [5] . In this method, electrochemically active elements are selectively removed by chemical reactions or thermal melting processes, producing nanostructured metal architectures. Potential drawbacks to this method can include disordered porosity, slow chemical reactions, high temperatures and toxic or corrosive processing chemistries. Alternative methods using organic ligands or capping agents have been developed to control Ag nanostructures. Here, organic ligands such as myristic acid or alkanethiol are bound at nanoparticle surfaces to prevent Ag particle aggregation, generally producing very monodispersive spherical particles [6] , [7] . Capping agents such as poly(vinyl pyrrolidone) may be used to modify seed crystal surface to enable growth of oriented Ag nanorods and nanowires [8] . Poly(vinyl pyrrolidone is understood to preferentially interact with specific nanocrystal surfaces such as {100} to inhibit growth of that orientation, compared with other crystal faces, enabling in oriented one- to two-dimensional (1–2D) Ag nanostructures. A mild ‘etching’ process and galvanic replacement method using silver nanocubes as sacrificial templates has demonstrated hollow nanostructure synthesis [2] . Galvanic replacement may be further combined with processes such as co-reduction and the Kirkendall effect to produce more complex nanostructures and/or compositional control [1] . Other effective chemical methods of 1D Ag nanorod production include templating of fast reaction kinetics [9] and block copolymer-directed growth and deposition on patterned substrates [10] . Many of these methods are enabled by the unique twinning behaviour of Ag particles and seed crystals, which enables definition of unusually faceted shapes through crystal nucleation and growth [2] . Many chemical methods use such defect structures (also the most reactive sites) to achieve oriented growth of Ag nanostructures; for example, oriented attachment was used to grow chain-like Ag nanostructures [11] . It has been shown elsewhere that an external stress induced by high-pressure compression can alter the mechanism of defect motion in atomic lattices through induced phase transformations [12] , [13] , [14] . Depending on the pressure condition, different Ag phase and structural transformations were observed: under hydrostatic pressure up to 10 GPa, Ag nanoparticles with sizes of 5–10 nm underwent a reversible, linear, pressure-dependent structural transformation [14] . At higher uniaxial compressions, disordered Ag microstructure was rearranged through phase transformations to form Ag nanoparticles with much higher stiffness [12] , [13] , [15] . Recent transmission electron microscopy (TEM) studies further confirmed these phase transformations in Ag microstructures and proposed that external stress can effectively alter the defect mode of Ag microstructures through relaxation of surface and internal strain [15] , [16] . These mechanisms suggest mechanical routes may both manipulate the size and shape of Ag nanostructures, as well as enhance the mechanical stability of resultant 1D nanostructures. Here we describe a mechanical compression method using a diamond anvil cell (DAC) to synthesize Ag nanostructures through pressure-directed assembly, with concurrent sintering of spherical Ag nanoparticles into nanowires. In this method, ordered Ag nanoparticle arrays were loaded into a DAC at ambient pressure, and subjected to compressive stresses of 0–15 GPa to induce array compression and ultimately phase transformation-induced nanowire sintering. Through in-situ high-pressure small angle X-ray scattering (HP-SAXS) and high-resolution TEM (HR-TEM) studies, it was observed that up to an external pressure of 8 GPa, the unit cell dimension of ordered Ag nanoparticle arrays could be systematically and reversibly manipulated. This allowed fine-tuning of interparticle separation distance and in-situ demonstration of reversible Ag surface plasmonic resonance (SPR) frequency. Consolidation of these arrays into Ag nanorods and nanowires was observed for external pressures >8 GPa, via stress-induced sintering of the spherical nanoparticle arrays. HR-TEM imaging shows that each Ag nanowire consists of individual Ag particle crystal domains with an interconnected zigzag morphology, suggesting orientation-directed sintering. Twinning faults within sintered Ag nanowires were clearly observed, which confirms that the Ag networks are formed by direct sintering of individual spherical nanoparticles. We found that exposure of specific Ag nanoparticle crystal surfaces and presence of particular grain boundaries facilitated the interesting mechanical synthesis process. Investigation through high-pressure, wide angle X-ray scattering (HP-WAXS) in combination with theoretical computations shows that high-pressure-induced stress can both effectively refine Ag microstructures and potentially manipulate the mechanical stability of Ag nanostructures. It is believed the fabrication process is potentially a facile method of 1D nanostructure development without the need for thermal processing, chemical reaction or removal of reaction byproducts. Ag nanoparticle array before mechanical compression Ag nanoparticles were synthesized through a thermal decomposition method using myristic acid as surface ligand [6] . 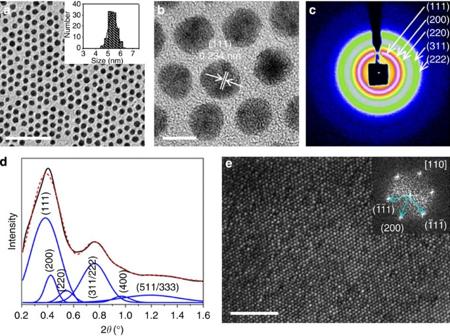Figure 1: Representative electron microscopy images of monodispersive silver nanoparticles used in the stress-induced sintering processes. (a) TEM image of the monodispersive silver nanoparticles. Inset shows the size distribution of the silver nanoparticles. (b) A representative HR-TEM image of the silver nanoparticles with [110] orientation. (c) A typical HP-SAXS image of the ordered Ag nanoparticle arrays loaded in DAC at ambient pressure. (d) The SAXS pattern integrated fromcwith fitted peaks. The theoretical fitting curve (red-dashed line) further confirms fcc symmetry. The solid blue curves present the Bragg reflections of each diffraction plane specified by Miller indices (hkl) that are characteristic of an fcc mesophase with space group ofFmm(the calculated unit cell parametera=120.5 Å). The relative weak intensity of (220) peak is due to the preferred orientation along [110] direction. (e) Representative plan-view SEM image of an ordered Ag nanoparticle array. Inset shows the Fast-Fourier transform from the image in (e). The scale bars in (a), (b) and (e) represent 50, 5 and 100 nm, respectively. Figure 1 shows a representative TEM image and size distribution of the Ag nanoparticles used in this study. The Ag nanoparticles are fairly monodisperse with an average diameter of 5.5 nm and a narrow size distribution ( Fig. 1a , inset). The HR-TEM image in Fig. 1b shows that these nanoparticles are crystalline with faceted surfaces. The Ag nanoparticles display five-fold twinning morphology with surface termination of (111) facets. Figure 1: Representative electron microscopy images of monodispersive silver nanoparticles used in the stress-induced sintering processes. ( a ) TEM image of the monodispersive silver nanoparticles. Inset shows the size distribution of the silver nanoparticles. ( b ) A representative HR-TEM image of the silver nanoparticles with [110] orientation. ( c ) A typical HP-SAXS image of the ordered Ag nanoparticle arrays loaded in DAC at ambient pressure. ( d ) The SAXS pattern integrated from c with fitted peaks. The theoretical fitting curve (red-dashed line) further confirms fcc symmetry. The solid blue curves present the Bragg reflections of each diffraction plane specified by Miller indices (hkl) that are characteristic of an fcc mesophase with space group of Fm m (the calculated unit cell parameter a =120.5 Å). The relative weak intensity of (220) peak is due to the preferred orientation along [110] direction. ( e ) Representative plan-view SEM image of an ordered Ag nanoparticle array. Inset shows the Fast-Fourier transform from the image in ( e ). The scale bars in ( a ), ( b ) and ( e ) represent 50, 5 and 100 nm, respectively. Full size image The measured lattice fringe 0.234 nm corresponds to a (111) spacing. Through a solvent evaporation process, described in the Methods section, these nanoparticles self-assembled into highly ordered superlattices. Figure 1c,d show the SAXS patterns of ordered nanoparticle arrays loaded in a DAC without pressurization. The SAXS image and integrated pattern collected at ambient pressure indicate a superlattice structure specific to a face-centred-cubic (fcc) mesophase with space group Fm m . The nanoparticle assembly exhibits a preferred orientation with (110) planes parallel to the substrate, which is normal to incident X-rays after mounting the sample-loaded DAC on the stage. The unit cell parameter a is calculated to be 120.5 Å. Figure 1e shows a representative plan-view scanning electron microscopy (SEM) image, confirming the [110] orientation. Fast-Fourier transform ( Fig. 1e , inset) analyses confirm that Ag nanoparticles are organized in a periodically ordered fcc mesophase with a preferred [110] orientation. Stress-induced formation of Ag nanowires The pressure in DAC was monitored using the pressure-dependent ruby fluorescent method (ruby R 1 line) [17] . HP-SAXS and HP-WAXS measurements, in combination with TEM studies, were carried out on Ag nanoparticle arrays over a pressure range of 0–15 GPa. 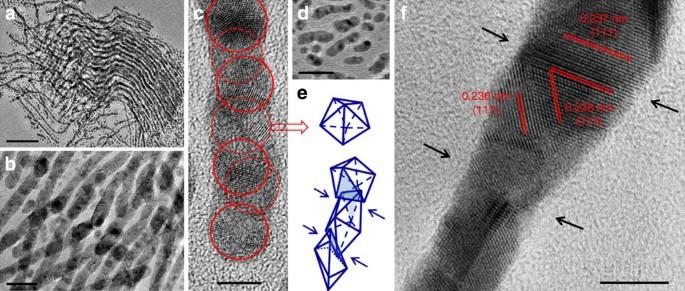Figure 2: Representative TEM images of Ag nanostructures synthesized under high-pressure-induced mechanical sintering of spherical Ag nanoparticle arrays. (a) A bundle of Ag nanowires. (b) HR-TEM image of reassembled nanowires after solvent evaporation. (c) HR-TEM image of a single Ag nanowire showing the zigzag morphology and twinning microstructure. Red circles are used for guidance of viewing individual crystal domains made up of Ag nanoparticles. Solid circles show the images close to the view direction, while dash circles show those further away from the view direction. (d) Ag nanorods. (e) Schematic of five-fold twinning microstructures and oriented sintering through (111) attachment evident in the HR-TEM image inf. (f) HR-TEM image of a single Ag nanowire showing oriented crystal sintering. Scale bars, 100, 20, 5, 20 and 5 nm (a–f, respectively). Figure 2a,b show the representative TEM images of 1D Ag nanostructures after pressure was released to ambient (amb) conditions. The resulting Ag nanowire array consists of individual Ag nanowires with a 2D hexagonal (hex) packing. These nanowire arrays were collected from the DAC and then dissolved in organic solvents such as toluene to form stable colloidal suspensions. The wires produced were uniform in diameter and length, and had an average diameter of 7.6 nm with an s.d. of 10%. HR-TEM imaging ( Fig. 2b,c,f ) reveals that the Ag nanowires are polycrystalline with an apparent twinning feature. Along the c axis, each nanowire consists of crystalline nanodomains that have domain sizes close to that of the original spherical Ag nanoparticles. This suggests that the Ag nanowires were developed through direct sintering of spherical Ag nanoparticles along the c axis. Detailed HR-TEM studies confirm that Ag nanoparticles are sintered through specific (111) to (111) facet surface interactions ( Fig. 2c,f ). Owing to such oriented sintering, the final Ag nanowires display a typical zigzag surface morphology, as proposed in Fig. 2e . We believe the increase of the nanowire diameter (7.6 nm) in comparison with the original nanoparticle (5.5 nm) is likely to be caused by uniaxial compression along the nanowire c axis, as proposed in the subsequent discussion section. Figure 2: Representative TEM images of Ag nanostructures synthesized under high-pressure-induced mechanical sintering of spherical Ag nanoparticle arrays. ( a ) A bundle of Ag nanowires. ( b ) HR-TEM image of reassembled nanowires after solvent evaporation. ( c ) HR-TEM image of a single Ag nanowire showing the zigzag morphology and twinning microstructure. Red circles are used for guidance of viewing individual crystal domains made up of Ag nanoparticles. Solid circles show the images close to the view direction, while dash circles show those further away from the view direction. ( d ) Ag nanorods. ( e ) Schematic of five-fold twinning microstructures and oriented sintering through (111) attachment evident in the HR-TEM image in f . ( f ) HR-TEM image of a single Ag nanowire showing oriented crystal sintering. Scale bars, 100, 20, 5, 20 and 5 nm ( a – f , respectively). Full size image Stress-induced assembly of Ag nanoparticles and nanowires Integrated HP-SAXS and HP-WAXS patterns of Ag nanoparticle arrays provide direct experimental evidence about how increasing pressure governs nanoparticle assembly towards an ultimate formation of Ag nanowires. 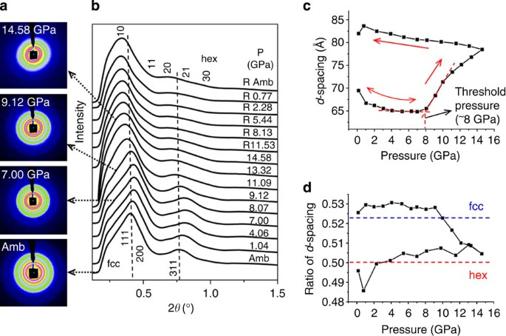Figure 3: Structural evolution of Ag nanoparticle arrays during high-pressure-induced assembly and sintering processes. (a) Representative HP-SAXS images of Ag nanoparticle arrays collected at ambient pressure (Amb or 0 GPa), 7 GPa, 9.12 GPa and 14.58 GPa. (b) The integrated spectra from the HP-SAXS images at varied pressures. (c) Thed-spacing changes of the first Bragg reflection along with the pressure in each HP-SAXS spectrum inb. (d)d-spacing ratioRat different pressures. Figure 3 shows the complex structural evolution of nanoparticle arrays during high-pressure-induced assembly and sintering processes. We observed two pressure-directed phase processes at distinct length scales, separated by a threshold pressure of ~\n8 GPa. Below 8 GPa, we observed a mesoscale pressure-directed assembly of Ag nanoparticle arrays. From ambient pressure to 8 GPa, the HP-SAXS patterns are consistent with the indexed fcc mesophase. TEM studies revealed that Ag nanoparticles were not sintered and still maintained the original spherical shape. Gradual shift of all the SAXS peaks to higher 2 θ (or lower d -spacing) ( Fig. 3a,b ) suggests a pressure-induced shrinkage of the nanoparticle superlattice. When pressure was gradually released from 8 GPa to ambient pressure, all the HP-SAXS peaks shifted back to their original positions, which indicates that the change of Ag superlattice dimension is reversible between atmospheric pressure and 8 GPa. This reversible behaviour was further verified by the d -spacing changes ( Fig. 3c ) and the constant d -spacing ratio R at varied pressure ( Fig. 3d ). Below 8 GPa, R remained the same and close to the theoretical value R (for example, the ratio of d -spacing of the second to the first major peak)= for an fcc superlattice. The lattice constant a reduced from 120.5 Å at ambient pressure to 112.3 Å at 7 GPa and returned back to 120.5 Å when pressure was completely released. In this case, the interparticle separation distance along the [110] direction can be reversibly tuned between 85.2 and 79.4 Å. This reversible behaviour allows in situ investigation of pressure-tuned, reversible Ag nanoparticle SPR behaviour versus interparticle spacing. Figure 3: Structural evolution of Ag nanoparticle arrays during high-pressure-induced assembly and sintering processes. ( a ) Representative HP-SAXS images of Ag nanoparticle arrays collected at ambient pressure (Amb or 0 GPa), 7 GPa, 9.12 GPa and 14.58 GPa. ( b ) The integrated spectra from the HP-SAXS images at varied pressures. ( c ) The d -spacing changes of the first Bragg reflection along with the pressure in each HP-SAXS spectrum in b . ( d ) d -spacing ratio R at different pressures. Full size image Stress-induced structural rearrangement A second phase, structural rearrangement process, which starts at 8 GPa and finishes at 15 GPa, is consistent with a phase transformation of the nanoparticle array and resulting uniaxial particle consolidation. In the intermediate stage from 8 to 15 GPa, the overall particle lattice was distorted and could not be simply indexed in either an fcc or a 2D hexagonal mesophase. R varied between 0.522 and 0.5. After release of the applied pressure, the HP-SAXS patterns were consistent with a 2D hexagonal mesophase, in which R =( d 20 / d 10 ) becomes ~\n0.5, which is both equal to the theoretical ratio d 20 / d 10 for a 2D hexagonal mesophase, and consistent with the HP-SAXS indexing and TEM results. During the second phase transformation, we observed a reversible atomic structural distortion within the Ag nanoparticles. At ambient pressure, the atomic lattice of Ag nanoparticles exhibited a cubic crystal microstructure. On increase of pressure to 14.28 GPa, all WAXS peaks shifted to higher angle. This pressure-induced decrease of d -spacing indicates an apparent shrinkage of lattice dimension ( Fig. 4a ). After release of pressure back to ambient pressure, all the HP-WAXS peaks shifted back to the original positions. Thus, the overall phase transformation process was reversible. This was also confirmed by the fact that both the increase and decrease of d 111 spacing in the pressure circle follow the same linear pathway ( Fig. 4b ). It is interesting to note that after compression, the WAXS patterns became much more intense ( Fig. 4c ), indicative of increased number of atomic planes or crystalline coherence. This observation suggests that high-pressure compression may refine the Ag microstructure. 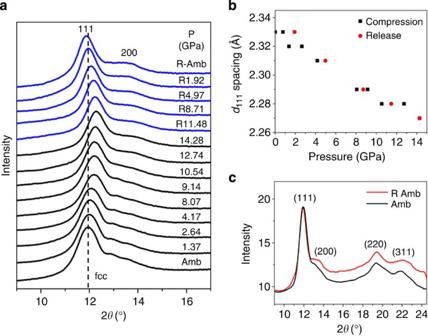Figure 4: Microstructural evolution of Ag nanoparticles (atomic lattice) during high-pressure-induced assembly and sintering processes. (a) Representative HP-WAXS patterns collected at various pressures. (b) The change ofd111spacing as a function of pressure. (c) Integrated HP-WAXS patterns of Ag nanoparticles before (black) and after (red) the pressure was released to ambient condition. Figure 4: Microstructural evolution of Ag nanoparticles (atomic lattice) during high-pressure-induced assembly and sintering processes. ( a ) Representative HP-WAXS patterns collected at various pressures. ( b ) The change of d 111 spacing as a function of pressure. ( c ) Integrated HP-WAXS patterns of Ag nanoparticles before (black) and after (red) the pressure was released to ambient condition. Full size image Mechanical property As discussed here and in previous work [12] , [13] , [14] , [15] , [16] , [18] , high-pressure stress can effectively induce Ag microstructure phase transformations and potentially manipulate the mechanical stability of Ag nanoparticles. Gu et al. [12] found an unexpected high stiffness of Ag and gold (Au) nanoparticles under high pressure. In our studies, we found that Ag nanoparticles exhibit a threshold pressure of 8 GPa. We used the Vinet (equation (1)) and the third-order Birch–Murnaghan (B–M) equation of states (equation (2)) to extract the effective bulk moduli for Ag nanoparticles. In the equations, B 0 is the ambient pressure bulk modulus, B 0 ′ is the pressure derivative of the bulk modulus ( B 0 ′=dB 0 /dP ), V is the unit cell volume under pressure and V 0 is the initial unit cell volume at ambient pressure. Based on the experimental compression curves (volume versus pressure in Fig. 5 ), the fitted bulk modulus of Ag is 57.1 GPa from the Vinet equation of state (equation (1)) and 44.2 GPa from the third-order B–M equation of state (equation (2)). 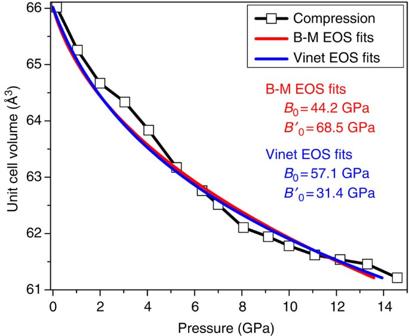Figure 5: Calculation of bulk modulus. Experimental compression curve for Ag (volume as a function of pressure) and the calculated bulk modules from fitting of Birch–Murnaghan and Vinet’s equation of state. Figure 5: Calculation of bulk modulus. Experimental compression curve for Ag (volume as a function of pressure) and the calculated bulk modules from fitting of Birch–Murnaghan and Vinet’s equation of state. Full size image Stress-induced optical coupling As discussed above, the high-pressure compression allows reversible manipulation of structural parameters of nanoparticle superlattices such as interparticle distance ( Fig. 3 ) during compression and release. This provides unique robustness for in-situ and reversible interrogation of both chemical and physical coupling interactions that depend on interparticle distance in nanoparticle assemblies, which has not normally been feasible for top-down and bottom-up fabrication methods [19] . We observed a tunable SPR of Ag nanoparticles and nanowires depending on external compression and release of pressure ( Fig. 6 ). At ambient pressure, the ultraviolet–visible spectrum shows a single peak at 518 nm corresponding to the Ag nanoparticle assemblies. Significant red shifts from 518 to 548 nm were observed on increasing pressure. Based on the TEM and HP-SAXS results ( Fig. 3c,d ), the Ag nanoparticles are not sintered before 8 GPa. Thus, we infer the red shift is due to inter-nanoparticle interactions (or SPR) as the interparticle distance becomes smaller on increase of the external pressure ( Fig. 3c ). We observed that below 8 GPa, SPR spectra shifted back to the original peak position when pressure was completely released. Thus, the SPR appears to be reversibly tuned by pressure. Above 8 GPa, we observed a new SPR peak corresponding to the formation of nanorods and nanowires, and their interactions. According to the TEM and HP-SAXS results, Ag nanoparticles start to contact each other and sinter into nanorods and nanowires at pressures above 8 GPa. The corresponding SPR spectra displayed a gradual blue shift from 548 to 523 nm, indicative of the gradual formation of nanorods and their growth to nanowires from 8 to 15 GPa. When the pressure was released, the SPR peak red shifted to 556 nm, which we infer is consistent with the de-aggregation of nanowires with decreased pressure. 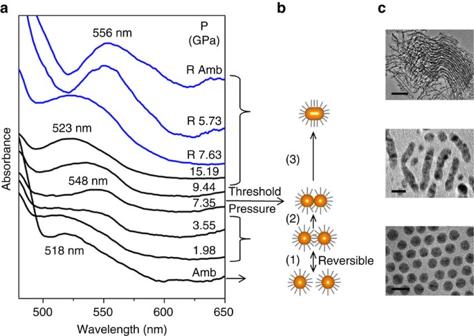Figure 6: Structure–property correlation of Ag nanoparticles superlattice during high-pressure compression and release. (a)In-situultraviolet–visible spectra of thin films of ordered Ag nanoparticles superlattice. (b) Schematic of nanoparticle assembly and sintering under high pressure: (1) below 8 GPa, nanoparticle superlattices shrink and spring back reversibly; (2) at the threshold pressure of 8 GPa, nanoparticles contact, driven by high pressure and start to sinter; (3) above 8 GPa, nanoparticles sinter and form nanorods and nanowires depending on applied pressure. (c) TEM images of Ag corresponding nanostructures to different stages of Ag nanoparticle aggregation inband optical signature ina. Scale bars, 100, 10 and 10 nm (c, from top to bottom). Figure 6: Structure–property correlation of Ag nanoparticles superlattice during high-pressure compression and release. ( a ) In-situ ultraviolet–visible spectra of thin films of ordered Ag nanoparticles superlattice. ( b ) Schematic of nanoparticle assembly and sintering under high pressure: (1) below 8 GPa, nanoparticle superlattices shrink and spring back reversibly; (2) at the threshold pressure of 8 GPa, nanoparticles contact, driven by high pressure and start to sinter; (3) above 8 GPa, nanoparticles sinter and form nanorods and nanowires depending on applied pressure. ( c ) TEM images of Ag corresponding nanostructures to different stages of Ag nanoparticle aggregation in b and optical signature in a . Scale bars, 100, 10 and 10 nm ( c , from top to bottom). Full size image The strong plasmonic resonance of metal nanoparticles depends significantly on the interparticle spacing [20] . When nanoparticle spacing is decreased, direct near-field coupling of light between nanoparticles gives rise to resonant collective electron plasmonic oscillation, leading to a red shift of the SPR peak. In our case, the Ag nanoparticles spacing is reversibly tuned via external high-pressure compression. Below 8 GPa, the hydrostatic pressure drives the nanoparticle lattice structure to shrink, causing gradual approach of nanoparticles along with applied pressure as shown in Fig. 3b,c . Hence, the external pressure leads to smaller interparticle spacing and enables stronger local inter-nanoparticle interactions, consistent with a red shift of the SPR peak (shown in Fig. 6 ). When the external pressure is released, the nanoparticle lattice structure is elastically relaxed and the interparticle spacing is observed to increase along with the pressure release, concomitant with return of the SPR peak position to its original atmospheric pressure value. Overall, the SPR is reversibly tuned in the pressure range of 0~\n8 GPa. For applied pressure larger than 8 GPa, nanoparticles were observed to sinter and consequently form 2D hexagonal arrays (or bundles) of Ag nanowires with a side-by-side arrangement. We believe that such extended side-by-side interactions enhance the longitudinal SPR mode, consistent with a blue shift of the SPR peak (from 548 to 523 nm, in Fig. 6 ) [20] , [21] , [22] . Careful analyses and reasonable correlations of in-situ SAXS and SPR measurements under pressure allow reconstruction of the mechanism by which external pressure drives Ag nanoparticle rearrangement into highly ordered 2D nanowire arrays ( Fig. 7 ). At ambient conditions, Ag nanoparticles pack into an fcc lattice with a preferred [110] orientation. The ordered nanoparticle arrays in a pressure medium of silicone oil were loaded into a DAC with [110] orientation to both the compression axis and incident X-rays. On initial hydrostatic compression, Ag nanoparticle arrays reduce lattice dimension linearly with pressure. Nanoparticles decreased separation but did not contact directly at pressures below 8 GPa. In this low-pressure circle of 0~\n8 GPa, Ag nanoparticle arrays maintained an fcc structure and displayed reversible pressure-dependent changes of compressibility and SPR. However, for pressures >8 GPa, the compression developed anisotropically, resulting in onset of uniaxial compression and radial expansion of nanoparticle arrays along with and normal to X-rays, respectively. Accordingly, nanoparticles are believed to contact directly along the X-ray direction and, simultaneously, surface ligands are displaced radially away from the uniaxial compression direction, thus expanding the inter-nanoparticle distance in the direction normal-to-uniaxial compression axis (that is, X-ray direction). Direct contact of nanoparticles caused a preliminary formation of nanorods and an associated blue shift of the SPR spectra. Continuing compression drives nanoparticle contacting with increasing area, resulting in an ultimate formation of long and stable nanowire arrays with a slightly increased diameter. The typical [110] orientation of nanoparticles along X-rays (that is, uniaxial compression axis) favours the development of a 2D hexagonal structure for the formed nanowire arrays. 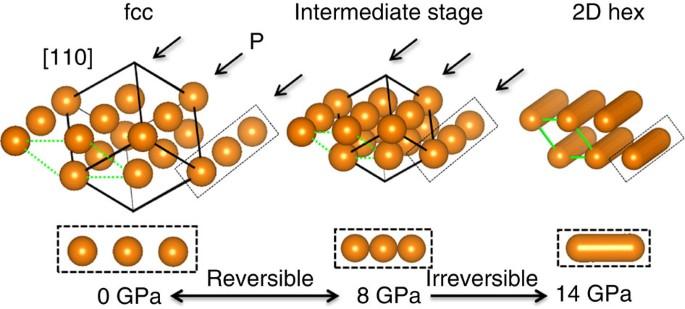Figure 7: Stress-induced assembly and sintering of nanoparticle superlattices. Reconstruction of the pressure-driven structure transformation pathway of Ag nanoparticles from three-dimensional packed fcc structure to 2D hexagonal nanowire arrays. Figure 7: Stress-induced assembly and sintering of nanoparticle superlattices. Reconstruction of the pressure-driven structure transformation pathway of Ag nanoparticles from three-dimensional packed fcc structure to 2D hexagonal nanowire arrays. Full size image In summary, high-pressure-directed assembly of nanoparticles and sintering enable both reversible tuning of structural parameters of nanoparticle superlattices for collective optical properties such as SPR, as well as for irreversible synthesis of 1D Ag nanostructures with a differing SPR signature. This method may represent a flexible approach for engineering of nanoparticle assemblies, reversible study of interparticle energy transfer and fabrication of new nanostructured materials. We expect the method to be applicable to a wide range of nanoparticle or building block compositions, including semiconductors (for example, CdSe) and magnetic nanostructures (for example, FePt) with further application to nanoelectronics and photonics. In general, exerting pressure-dependent control over the structure of nanoparticle arrays provides a flexible system to understand fundamental collective physical characteristics and to develop insight into novel electronic and photonic behaviours [19] . Synthesis of Ag nanoparticles and formation of ordered arrays Ag nanoparticles functionalized with myristate were synthesized using a literature method [6] . Briefly, silver myristate (C 13 H 27 CO 2 Ag, 2.0 g) suspended in triethylamine, NEt 3 (17.5 ml), was heated at 80 °C for 1.5 h under an Ar atmosphere. The resulted Ag nanoparticles were precipitated with acetone (20 ml). After centrifuging at 4,000 r.p.m. for 2 min, the precipitate was re-dispersed in toluene (2 ml) and precipitated with ethanol (20 ml). The Ag nanoparticles were collected after centrifugation and dried under vacuum for 10 min. Nanoparticle arrays were fabricated through a solvent evaporation method by drop-casting Ag nanoparticle solutions (100 mg ml −1 in toluene with 25% polystyrene) on a silicon wafer. A piece of the Ag nanoparticle film (~\n150 μm) was peeled off the silicon wafer and loaded into the DAC for in-situ HP-SAXS, HP-WAXS and absorption measurements. Characterization TEM study was performed on a JEOL 2010 with a 200-kV acceleration voltage, equipped with a Gatan slow scan charge-coupled device camera. SEM images were taken using a Hitachi S-5200 FEG microscope at 5 kV. Ultraviolet–visible spectra were obtained on a Perkin Elmer Lambda 950 spectrophotometer. In-situ HP-SAXS and HP-WAXS measurements were performed on the B1 station at the Cornell High Energy Synchrotron Source (CHESS) with a monochromatic X-ray radiation of wavelength λ =0.485946 Å [23] . The distance between the sample and a large area MAR345 detector was 727.19 mm, as determined using both CeO 2 and silver behenate powder standard. Several small ruby chips were loaded into the DAC chamber as inside pressure probes to monitor the sample pressure by a standard pressure-dependent ruby fluorescence technique [17] . Scattering images were calibrated and integrated using the Fit2D software. The scattering curves were fitted in Gaussian distribution using the Origin 8 programme. The in-situ ultraviolet–visible spectra of the ordered Ag nanoparticles superlattice thin film during high-pressure compression and release were measured by a PerkinElmer Lambda 950 ultraviolet–visible spectrometer. The DAC loaded with Ag nanoparticle film was inserted into the sample beam line, and a blank gasket with a 250-μm hole was inserted into the reference beam line. All other procedures were the same as regular procedures. How to cite this article: Li, B. et al. Stress-induced phase transformation and optical coupling of silver nanoparticle superlattices into mechanically stable nanowires. Nat. Commun. 5:4179 doi: 10.1038/ncomms5179 (2014).